Mitochondrial defects trigger proliferation of neighbouring cells via a senescence-associated secretory phenotype inDrosophila Cell–cell interactions play important roles in epithelial tumorigenesis. Here we show in Drosophila imaginal epithelium that Ras activation and mitochondrial dysfunction, frequent alterations in cancers, cause cellular senescence and senescence-associated secretory phenotype (SASP), which leads to overgrowth of neighbouring tissue. Ras-activated cells express several hallmarks of cellular senescence such as elevation of senescence-associated β-galactosidase activity, upregulation of the Cdk inhibitor Dacapo, heterochromatinization and cellular hypertrophy. Strikingly, defects in mitochondrial function cause Ras-activated cells to undergo DNA damage response, cell cycle arrest and thereby induce SASP, exhibiting full aspects of cellular senescence. Mechanistically, mitochondrial defects in conjunction with Ras cause production of reactive oxygen species, downregulation of CycE activity and activation of p53, which cooperate together to trigger a cell cycle arrest-Jun N-terminal kinase (JNK) feedback loop that amplifies JNK activation, leading to upregulation of the inflammatory cytokine Unpaired. Our data suggest that mitochondrial defects promote Ras-induced cellular senescence and thereby contribute to tumour progression through SASP. Cell–cell interactions within tumour microenvironment play a crucial role in epithelial cancer development. For instance, communication among oncogenic cells, stromal fibroblasts, immune cells and normal epithelial cells can drive tumour development and progression [1] . Although the mechanism by which oncogenic cells cooperate with surrounding cells to drive tumour progression is still elusive, recent studies have suggested that cellular senescence, the state of ultimate and irreversible cell cycle arrest, can promote cancer development through cell–cell communication. Cellular senescence is provoked by diverse cellular stresses such as chromosomal instability, telomere shortening, oxidative stress, DNA damage and aberrant activation of oncogenes [3] , [4] , [5] , [6] . The oncogene-induced cellular senescence has been shown to exert a tumour-suppressive effect by inducing cell cycle arrest in premalignant cells [3] , [4] , [6] . In fact, premalignant human nevi and colon adenomas contain cells exhibiting cellular senescence phenotypes, but senescent cells are markedly reduced in malignant melanomas and adenocarcinomas developed from these lesions [7] , [8] . In addition, in mouse models with activated Ras signalling or pten deletion, senescent cells are abundant in premalignant lesions but are scarce in cancers eventually developed [9] , [10] , [11] . These observations raise a question of how tumours eventually emerge from such heterogeneous oncogenic lesions with a significant population of senescent cells. Interestingly, recent studies in cell culture systems have revealed non-autonomous functions of senescent cells; cells undergoing cellular senescence secrete a variety of cytokines, chemokines and growth factors that affect surrounding cells, which is known as the senescence-associated secretory phenotype (SASP) or the senescence-messaging secretome [4] , [6] , [12] , [13] , [14] , [15] , [16] . Thus, in certain settings, cells exhibiting SASP could exert a tumour-promoting effect on their surrounding cells [15] , [17] . For instance, senescent fibroblasts secrete an epidermal growth factor-like growth factor amphiregulin and a cytokine growth-related oncogene-α, both stimulate proliferation of premalignant epithelial cells in cell culture systems [12] , [18] . In addition, some SASP factors such as interleukin-6 (IL-6) and IL-8 can promote malignant transformation in conjunction with activated oncogenes [19] , [20] , [21] . Furthermore, it has been shown in obesity mouse model that SASP factors play crucial roles in promoting development of obesity-associated hepatocellular carcinoma [22] . However, the molecular link between cellular senescence phenotypes and SASP, as well as the mechanism by which cellular senescence drives SASP induction in vivo, are poorly understood. Drosophila provides a powerful model system for studying cell–cell communication within developing epithelium through the genetic mosaic technique [23] . We have recently performed a genetic screen in Drosophila imaginal epithelium to identify genes that drive tumour progression through cell–cell interactions and found that mutations in mitochondrial respiratory complexes in Ras-activated cells (Ras V12 / mito −/− cells) induce tumour progression in their neighbouring benign tumours [24] . Ras V12 / mito −/− cells upregulate production of an inflammatory cytokine Unpaired (Upd, an IL-6 homologue) and thereby promote growth and malignancy of surrounding Ras-induced benign tumours, exhibiting marked similarity with SASP. Here we show in Drosophila imaginal epithelium that clones of cells activated Ras signalling express several markers of cellular senescence such as elevation of senescence-associated β-galactosidase (SA-β-gal) activity, upregulation of G1 cyclin-dependent kinase (Cdk) inhibitor Dacapo (Dap, a p21/p27 homologue), heterochromatinization and increased cell size (cellular hypertrophy). Intriguingly, despite the upregulated expression of Dap, Ras-activated cells do not undergo cell cycle arrest. We find that mitochondrial dysfunction causes Ras V12 -expressing cells to induce cell cycle arrest in G1 phase, thereby leading to SASP. Our data suggest that mitochondrial defect causes Ras-activated cells to undergo cellular senescence in vivo . Furthermore, we dissect the genetic pathway of cellular senescence-mediated tumour progression through SASP. Ras induces cellular senescence markers in Drosophila Aberrant activation of oncogenes such as Ras can induce cellular senescence in mammalian cells. However, it has been unclear whether the oncogene-induced cellular senescence can also be induced in invertebrates. We first examined whether aberrant activation of Ras signalling in Drosophila imaginal epithelium causes cellular senescence. We found that clones of cells expressing oncogenic Ras V12 in the eye imaginal disc indeed exhibited several cellular senescence markers such as elevated SA-β-gal activity ( Fig. 1a,b ), upregulation of a Cdk inhibitor Dacapo (Dap, a p21/p27 homologue; Fig. 1c,d , Supplementary Fig. 1a,b ), elevation of histone H3-K9 trimethylation (which is associated with the senescence-associated heterochromatin foci; Fig. 1e,f ) and upregulation of heterochromatin protein-1 (HP-1; which binds to methylated K9 of histone H3; Supplementary Fig. 1c,d ). In mammalian cell culture systems, cells undergoing cellular senescence exhibit enlarged and flattened cell morphology. Similarly, we found that cells activating Ras signalling in imaginal epithelium showed increased cell size (1.20±0.02, relative to wild-type cells of 1.00±0.02) ( Fig. 1g,h ). Thus, cells with elevated Ras signalling in Drosophila epithelium exhibit several hallmarks of cellular senescence. 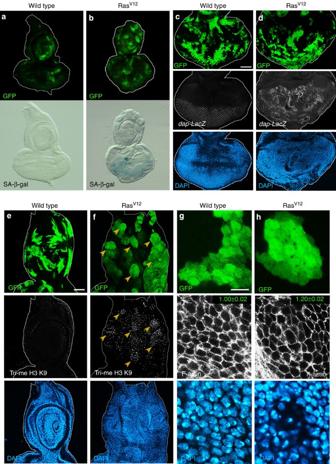Figure 1: Ras activation induces cellular senescence markers inDrosophila. (a,b) Eye-antennal disc bearing green fluorescent protein (GFP)-labelled wild-type (a) or RasV12(b) clones was subjected to SA-β-gal assay. (c,d) GFP-labelled wild-type (c) or RasV12(d) clones were induced indap-LacZeye-antennal disc and stained with anti-β-gal. (e,f) Eye-antennal disc bearing GFP-labelled wild-type (e) or RasV12(f) clones was stained with anti-Histone-H3-trimethyl-K9. Arrowheads indicate representative clones upregulating trimethylated Histone H3-K9. (g,h) Eye-antennal disc bearing GFP-labelled wild-type (g) or RasV12(h) clones was stained with phalloidin to visualize F-actin. Cell size was measured using ImageJ and was quantified as relative size to wild-type cells. Data were collected as mean±s.e., wild-type (n=186); RasV12(n=227). The nuclei were stained with 4',6-diamidino-2-phenylindole (DAPI). Scale bars, 50 μm (c,e) or 10 μm (g). SeeSupplementary Table 1for genotypes. Figure 1: Ras activation induces cellular senescence markers in Drosophila . ( a , b ) Eye-antennal disc bearing green fluorescent protein (GFP)-labelled wild-type ( a ) or Ras V12 ( b ) clones was subjected to SA-β-gal assay. ( c , d ) GFP-labelled wild-type ( c ) or Ras V12 ( d ) clones were induced in dap-LacZ eye-antennal disc and stained with anti-β-gal. ( e , f ) Eye-antennal disc bearing GFP-labelled wild-type ( e ) or Ras V12 ( f ) clones was stained with anti-Histone-H3-trimethyl-K9. Arrowheads indicate representative clones upregulating trimethylated Histone H3-K9. ( g , h ) Eye-antennal disc bearing GFP-labelled wild-type ( g ) or Ras V12 ( h ) clones was stained with phalloidin to visualize F-actin. Cell size was measured using ImageJ and was quantified as relative size to wild-type cells. Data were collected as mean±s.e., wild-type ( n =186); Ras V12 ( n =227). The nuclei were stained with 4',6-diamidino-2-phenylindole (DAPI). Scale bars, 50 μm ( c , e ) or 10 μm ( g ). See Supplementary Table 1 for genotypes. Full size image Mitochondrial defect causes Ras V12 cells to induce G1 arrest Cells undergoing cellular senescence exhibit an irreversible cell cycle arrest in G1 phase, which is one of the critical cellular events in cellular senescence. We thus examined whether clones of Ras-activated cells cause cell cycle arrest in G1 phase in imaginal disc using the cell cycle monitoring probe S/G2/M-Green [25] , [26] . Despite showing several phenotypic markers of cellular senescence ( Fig. 1 ), Ras V12 -expressing cells were not arrested in G1 phase, as most of these cells did not lose S/G2/M-Green expression ( Fig. 2a,b , quantified in Fig. 2e ). These results indicate that Ras activation is not sufficient for inducing all aspects of cellular senescence phenotypes and therefore Ras V12 -expressing cells are not senescent cells. These observations are consistent with previous reports in mammalian systems that SA-β-gal, increased cell size and senescence-associated heterochromatin foci are neither necessary nor sufficient for induction of cellular senescence [27] , [28] , [29] , [30] . Intriguingly, we found that, when mitochondrial respiratory function was simultaneously downregulated in Ras V12 -expressing cells (by introducing the mitochondrial respiratory complex I mutation Pdsw −/− ), such mutant cells caused cell cycle arrest in G1 phase ( Fig. 2d , quantified in Fig. 2e ), whereas cells with mitochondrial dysfunction alone only slightly suppressed cell cycle progression ( Fig. 2c , quantified in Fig. 2e ). Similarly, by introducing the Pdsw −/− mutation or the mitochondrial respiratory complex IV mutation CoVa −/− (hereafter, Pdsw −/− and CoVa −/− are referred to as mito −/− ), we have recently found that mitochondrial dysfunction in Ras V12 -expressing cells (Ras V12 / mito −/− cells) exhibit SASP-like phenotype, as such mutant cells upregulate production of the IL-6 homologue Upd, although cells expressing Ras V12 alone do not [24] . In addition, Ras V12 / mito −/− cells, but not Ras V12 cells or mito −/− cells, exhibited intranuclear foci of phosphorylated histone H2A variant (γH2Av; Fig. 2f-j ), an indicator of DNA damage response that plays a crucial role in the induction of cellular senescence [31] , [32] , [33] , [34] and SASP [35] , [36] . Furthermore, mitochondrial defect strongly enhanced cellular hypertrophy in Ras V12 -expressing cells (1.93±0.03, relative to wild-type cells of 1.00±0.02; Fig. 2l ), whereas mitochondrial dysfunction alone did not affect cell size (0.97±0.01, relative to wild-type cells of 1.00±0.02; Fig. 2k ). These results indicate that mitochondrial dysfunction causes Ras-activated cells to induce cellular senescence. Indeed, Ras V12 / mito −/− cells showed all other characters of cellular senescence observed in Ras V12 -expressing cells such as SA-β-gal activity, upregulation of p21/p27/Dap, histone H3-K9 trimethylation and upregulation of HP-1, whereas mitochondrial dysfunction alone did not induce such changes ( Supplementary Fig. 2a–n ). 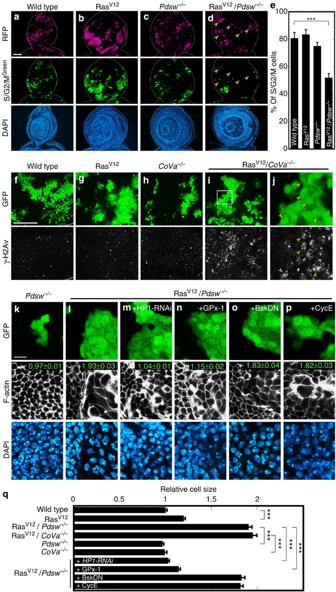Figure 2: Mitochondrial defect causes RasV12cells to undergo G1 arrest and cellular hypertrophy. (a–d) Eye-antennal disc bearing RFP-labelled wild-type (a), RasV12(b),Pdsw−/−(c) or RasV12/Pdsw−/−(d) clones was induced in S/G2/M-Green eye-antennal disc. Arrowheads indicate representative clones lacking S/G2/M-Green expression. (e) Quantification of % of S/G2/M-Green-positive cells in each clone. Five to eight imaginal discs were examined using ImageJ. S/G2/M-Green-positive cells were significantly fewer in RasV12/Pdsw−/−clones. Data were collected as mean±s.e., wild type (n=5); RasV12(n=5);Pdsw−/−(n=8); RasV12/Pdsw−/−(n=5). Student’st-test, ***P<0.0001. (f–j) Eye-antennal disc bearing green fluorescent protein (GFP)-labelled wild-type (f), RasV12(g),CoVa−/−(h) or RasV12/CoVa−/−(i,j) clones was stained with anti-γ-H2Av. (j) High-magnification image of the boxed area ini. Arrowheads in indicate cells exhibiting typical intranuclear γ-H2Av foci. (k–p) Eye-antennal disc bearing GFP-labelledPdsw−/−(k), RasV12/Pdsw−/−(l), RasV12/Pdsw−/−+HP1-RNAi (m), RasV12/Pdsw−/−+GPx-1 (n), RasV12/Pdsw−/−+BskDN(o) or RasV12/Pdsw−/−+CycE (p) clones was stained with phalloidin. (q) Cell size was measured using ImageJ and was quantified as relative size to wild-type cells. Data were collected as mean±s.e., wild-type (n=186); RasV12(n=227); RasV12/Pdsw−/−(n=339); RasV12/CoVa−/−(n=194);Pdsw−/−(n=103);CoVa−/−(n=99); RasV12/Pdsw−/−+HP1-RNAi (n=335); RasV12/Pdsw−/−+GPx-1 (n=167); RasV12/Pdsw−/−+BskDN(n=188); RasV12/Pdsw−/−+CycE (n=180). Student’st-test, ***P<0.0001. The nuclei were stained with 4',6-diamidino-2-phenylindole (DAPI). Scale bars, 50 μm (a,f) or 10 μm (k). SeeSupplementary Table 1for genotypes. Figure 2: Mitochondrial defect causes Ras V12 cells to undergo G1 arrest and cellular hypertrophy. ( a – d ) Eye-antennal disc bearing RFP-labelled wild-type ( a ), Ras V12 ( b ), Pdsw −/− ( c ) or Ras V12 / Pdsw −/− ( d ) clones was induced in S/G2/M-Green eye-antennal disc. Arrowheads indicate representative clones lacking S/G2/M-Green expression. ( e ) Quantification of % of S/G2/M-Green-positive cells in each clone. Five to eight imaginal discs were examined using ImageJ. S/G2/M-Green-positive cells were significantly fewer in Ras V12 / Pdsw −/− clones. Data were collected as mean±s.e., wild type ( n =5); Ras V12 ( n =5); Pdsw −/− ( n =8); Ras V12 / Pdsw −/− ( n =5). Student’s t -test, *** P <0.0001. ( f – j ) Eye-antennal disc bearing green fluorescent protein (GFP)-labelled wild-type ( f ), Ras V12 ( g ), CoVa −/− ( h ) or Ras V12 / CoVa −/− ( i , j ) clones was stained with anti-γ-H2Av. ( j ) High-magnification image of the boxed area in i . Arrowheads in indicate cells exhibiting typical intranuclear γ-H2Av foci. ( k – p ) Eye-antennal disc bearing GFP-labelled Pdsw −/− ( k ), Ras V12 / Pdsw −/− ( l ), Ras V12 / Pdsw −/− +HP1-RNAi ( m ), Ras V12 / Pdsw −/− +GPx-1 ( n ), Ras V12 / Pdsw −/− +Bsk DN ( o ) or Ras V12 / Pdsw −/− +CycE ( p ) clones was stained with phalloidin. ( q ) Cell size was measured using ImageJ and was quantified as relative size to wild-type cells. Data were collected as mean±s.e., wild-type ( n =186); Ras V12 ( n =227); Ras V12 / Pdsw −/− ( n =339); Ras V12 / CoVa −/− ( n =194); Pdsw −/− ( n =103); CoVa −/− ( n =99); Ras V12 / Pdsw −/− +HP1-RNAi ( n =335); Ras V12 / Pdsw −/− +GPx-1 ( n =167); Ras V12 / Pdsw −/− +Bsk DN ( n =188); Ras V12 / Pdsw −/− +CycE ( n =180). Student’s t -test, *** P <0.0001. The nuclei were stained with 4',6-diamidino-2-phenylindole (DAPI). Scale bars, 50 μm ( a , f ) or 10 μm ( k ). See Supplementary Table 1 for genotypes. Full size image SASP and cellular hypertrophy are separable processes Although there have been several studies on the mechanism by which senescent cells induce SASP factors, it is still unclear how the cellular senescence phenotypes are linked to SASP induction. We therefore sought to identify the molecules that link cellular senescence markers to SASP. When HP-1 expression was reduced by HP-1-RNAi in Ras V12 / mito −/− clones, cellular hypertrophy was almost completely abolished, placing cellular hypertrophy downstream of heterochromatin formation ( Fig. 2m , quantified in Fig. 2q ). However, blocking of both HP-1 expression and cellular hypertrophy did not suppress induction of non-autonomous overgrowth ( Supplementary Fig. 2o , quantified in Supplementary Fig. 2p ), suggesting that SASP and cellular hypertrophy are separable processes in cellular senescence. It has been shown that Ras V12 / mito −/− cells upregulate Upd through production of reactive oxygen species (ROS) and subsequent Jun N-terminal kinase (JNK) activation [24] . We found that blocking oxidative stress by overexpression of glutathione peroxidase (GPx-1) in Ras V12 / mito −/− clones significantly suppressed cellular hypertrophy, whereas blocking JNK signalling by Bsk DN did not affect the hypertrophy ( Fig. 2n,o , quantified in Fig. 2q ). Importantly, expression of either GPx-1 or Bsk DN in Ras V12 / mito −/− clones abolished non-autonomous overgrowth [24] . These data indicate that two cellular senescence markers, heterochromatinization and oxidative stress, are required for cellular hypertrophy, but the cellular hypertrophy is not essential for SASP induction. G1 cell cycle arrest is required for SASP We then sought to identify other cellular senescence markers responsible for SASP induction. Our genetic data so far presented indicate that mitochondrial dysfunction causes Ras-activated cells to undergo cellular senescence by inducing G1 arrest and SASP, suggesting the possible molecular link between cell cycle arrest and SASP induction. Strikingly, overexpression of CycE, which counters the function of p21/p27/Dap and promotes the G1/S transition, in Ras V12 / mito −/− clones significantly suppressed non-autonomous overgrowth ( Fig. 3a,b , Supplementary Fig. 3a–c , quantified in Supplementary Fig. 3g,h ). Furthermore, overexpression of CycE blocked induction of upd expression ( Fig. 3c , compare with Supplementary Fig. 3d ) as well as its upstream JNK activation (visualized by the puc-lacZ reporter [37] , [38] ; Fig. 3d , compare with Supplementary Fig. 3e ), both of which are essential for the induction of non-autonomous overgrowth by Ras V12 / mito −/− clones [24] . In contrast, overexpression of CycE had no effect on the induction of oxidative stress (as visualized by the gstD-GFP reporter [39] ; Fig. 3e , compare with Supplementary Fig. 3f ), which acts upstream of JNK activation in this signalling [24] , as well as the induction of cellular hypertrophy ( Fig. 2p , quantified in Fig. 2q ). These data suggest that cell cycle arrest is required for SASP induction at the downstream of oxidative stress. Indeed, we found that forced induction of G1 arrest by loss of cycE causes Ras V12 -expressing clones to induce non-autonomous overgrowth ( Fig. 3f ), whereas clones with cycE mutation alone do not ( Fig. 3g ). Similar to the case of Ras V12 / mito −/− clones, the non-autonomous overgrowth caused by Ras V12 / cycE −/− clones was suppressed by blocking JNK signalling ( Fig. 3h , quantified in Supplementary Fig. 3i ) or Yki activity ( Fig. 3i , quantified in Supplementary Fig. 3j ), a transcriptional co-activator that induces upd expression in Ras V12 / mito −/− clones [24] . Indeed, Ras V12 / cycE −/− clones exhibited JNK activation ( Fig. 3l ) and Upd induction ( Fig. 3n ), whereas Ras V12 alone or cycE mutation alone caused neither of them ( Fig. 3k,m , and data not shown) [24] . We also found that a reduction in Rb gene, a cell cycle inhibitor that is negatively regulated by CycE, significantly suppressed non-autonomous overgrowth caused by Ras V12 / mito −/− clones ( Fig. 3j , quantified in Supplementary Fig. 3k ). Together, these data indicate that cell cycle arrest in G1 phase causes Ras-activated cells to induce SASP. 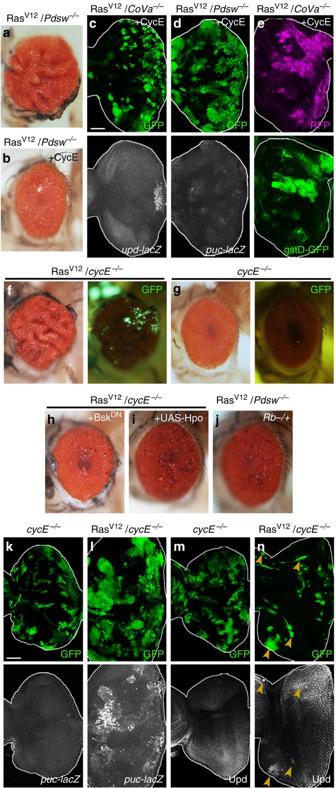Figure 3: Cell cycle arrest is required for inducing SASP. (a,b) Adult eye bearing RasV12/Pdsw−/−(a) or RasV12/Pdsw−/−+CycE (b) clones. SeeSupplementary Fig. 3afor wild-type eye. (c) Green fluorescent protein (GFP)-labelled RasV12/CoVa−/−+CycE clones were induced inupd-LacZeye-anntenal disc and stained with anti-β-gal. Endogenousupd-LacZexpression is indicated (c′, asterisk). (d) GFP-labelled RasV12/Pdsw−/−+CycE clones were induced inpuc-LacZeye-anntenal disc and stained with anti-β-gal. (e) RFP-labelled RasV12/CoVa−/−+CycE clones were induced ingstD-GFPeye-antennal disc. (f–j) Adult eye bearing GFP-labelled RasV12/cycE−/−(f),cycE−/−(g), RasV12/cycE−/−+BskDN(h), RasV12/cycE−/−+Hpo (i) or RasV12/Pdsw−/−,Rb/+ (j) clones is shown. (k,l) GFP-labelledcycE−/−(k) or RasV12/cycE−/−(l) clones were induced inpuc-LacZeye-anntenal disc and stained with anti-β-gal. (m,n) Eye-antennal disc bearing GFP-labelledcycE−/−(m) or RasV12/cycE−/−(n) clones was stained with anti-Upd. Arrowheads indicate representative clones upregulating Upd. Scale bars, 50 μm. SeeSupplementary Table 1for genotypes. Figure 3: Cell cycle arrest is required for inducing SASP. ( a , b ) Adult eye bearing Ras V12 / Pdsw −/− ( a ) or Ras V12 / Pdsw −/− +CycE ( b ) clones. See Supplementary Fig. 3a for wild-type eye. ( c ) Green fluorescent protein (GFP)-labelled Ras V12 / CoVa −/− +CycE clones were induced in upd-LacZ eye-anntenal disc and stained with anti-β-gal. Endogenous upd-LacZ expression is indicated ( c ′, asterisk). ( d ) GFP-labelled Ras V12 / Pdsw −/− +CycE clones were induced in puc-LacZ eye-anntenal disc and stained with anti-β-gal. ( e ) RFP-labelled Ras V12 / CoVa −/− +CycE clones were induced in gstD-GFP eye-antennal disc. ( f – j ) Adult eye bearing GFP-labelled Ras V12 / cycE −/− ( f ), cycE −/− ( g ), Ras V12 / cycE −/− +Bsk DN ( h ), Ras V12 / cycE −/− +Hpo ( i ) or Ras V12 / Pdsw −/− , Rb /+ ( j ) clones is shown. ( k , l ) GFP-labelled cycE −/− ( k ) or Ras V12 / cycE −/− ( l ) clones were induced in puc-LacZ eye-anntenal disc and stained with anti-β-gal. ( m , n ) Eye-antennal disc bearing GFP-labelled cycE −/− ( m ) or Ras V12 / cycE −/− ( n ) clones was stained with anti-Upd. Arrowheads indicate representative clones upregulating Upd. Scale bars, 50 μm. See Supplementary Table 1 for genotypes. Full size image Cell cycle arrest amplifies JNK signalling The fact that overexpression of CycE blocks JNK activation in Ras V12 / mito −/− cells raised the possibility that JNK signalling is activated through cell cycle arrest. To examine this possibility, we first utilized a JNK-dependent cell death phenotype caused by overexpression of the tumour-necrosis factor ligand Eiger. Ectopic expression of Eiger in the posterior region of the eye disc by the GMR -Gal4 driver causes JNK-dependent cell death that leads to a small eye phenotype [40] ( Fig. 4a ). Significantly, co-expression of CycE suppressed the small eye phenotype induced by Eiger ( Fig. 4b ). Conversely, when the expression of CycE was reduced by cycE -RNAi, the small eye phenotype was significantly enhanced ( Fig. 4c ). Importantly, overexpression of CycE or cycE -RNAi did not affect significantly the eye morphology ( Fig. 4d–f ). We also found that although overexpression of Eiger or cycE -RNAi in undifferentiated eye disc cells by the eyeless -Gal4 driver did not affect eye morphology ( Fig. 4g,h ), co-expression of Eiger and cycE-RNAi in these cells caused small eye phenotype ( Fig. 4i ), which was cancelled by blocking JNK signalling ( Fig. 4j ). These results suggest that CycE negatively regulates JNK signalling activity. We thus directly confirmed this using the JNK kinase Hemipterous (Hep). Overexpression of a constitutively active form of Hep (Hep CA ) in the posterior region of the eye disc led to the activation of JNK in this area ( Fig. 4k ). Significantly, co-expression of CycE suppressed this JNK activation ( Fig. 4l ), confirming that CycE antagonizes JNK activation. These data suggest that cell cycle arrest enhances JNK activation. Intriguingly, we found that JNK activation also induces cell cycle arrest, as clones of cells expressing Hep CA abolished BrdU incorporation in the second mitotic wave in the eye disc ( Fig. 4m,n ), suggesting that cell cycle arrest and JNK activation forms a positive feedback loop that amplifies the signalling ( Fig. 4o ). To verify this model, we induced clones of cells co-expressing Ras V12 and Hep CA in the eye disc, which have been shown to cause non-autonomous overgrowth [41] ( Fig. 4p ). Strikingly, non-autonomous overgrowth caused by Ras V12 +Hep CA clones was strongly suppressed by co-expression of CycE ( Fig. 4q , quantified in Supplementary Fig. 4a ), but not by co-expression of antioxidant enzyme Catalase ( Fig. 4r , quantified in Supplementary Fig. 4b ), consistent with our findings that cell cycle arrest acts downstream of oxidative stress and upstream of JNK activation. Together, these data show that cells undergoing cellular senescence induce SASP through cell cycle arrest-mediated amplification of JNK signalling. 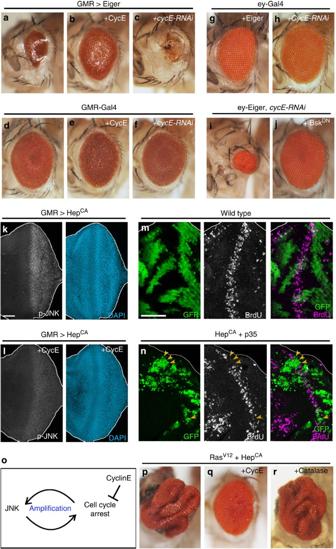Figure 4: Cell cycle arrest amplifies JNK activation. (a–j) Eye phenotypes ofGMR>Eiger (a),GMR>Eiger+CycE (b),GMR>Eiger+cycE-RNAi(c),GMR-Gal4 (d),GMR>CycE (e),GMR>cycE-RNAi(f),ey>Eiger (g),ey>cycE-RNAi(h), ey>Eiger+cycE-RNAi(i) andey>Eiger+cycE-RNAi+BskDN(j) are shown. (k,l) Eye disc expressing HepCA(k) or HepCA+CycE (l) in the posterior region (right half) was stained with anti-phospho-JNK antibodies. The nuclei were stained with 4',6-diamidino-2-phenylindole (DAPI). (m,n) 5-Bromodeoxyuridine (BrdU) labelling in eye disc bearing green fluorescent protein (GFP)-labelled wild-type (m) or HepCA+p35 (n) clones is shown. Arrowheads indicate second mitotic wave (SMW) cells lacking BdrU staining. (o) A model for the cell cycle arrest-JNK amplification loop in RasV12/mito−/−senescent cells. (p,q,r) Adult eye bearing RasV12+HepCA(p), RasV12+HepCA+CycE (q) or RasV12+HepCA+Catalase (r) clones is shown. Scale bars, 50 μm. SeeSupplementary Table 1for genotypes. Figure 4: Cell cycle arrest amplifies JNK activation. ( a – j ) Eye phenotypes of GMR >Eiger ( a ), GMR >Eiger+CycE ( b ), GMR >Eiger+ cycE-RNAi ( c ), GMR -Gal4 ( d ), GMR >CycE ( e ), GMR > cycE-RNAi ( f ), ey >Eiger ( g ), ey > cycE-RNAi ( h ) , ey >Eiger+ cycE-RNAi ( i ) and ey >Eiger+ cycE-RNAi +Bsk DN ( j ) are shown. ( k , l ) Eye disc expressing Hep CA ( k ) or Hep CA +CycE ( l ) in the posterior region (right half) was stained with anti-phospho-JNK antibodies. The nuclei were stained with 4',6-diamidino-2-phenylindole (DAPI). ( m , n ) 5-Bromodeoxyuridine (BrdU) labelling in eye disc bearing green fluorescent protein (GFP)-labelled wild-type ( m ) or Hep CA +p35 ( n ) clones is shown. Arrowheads indicate second mitotic wave (SMW) cells lacking BdrU staining. ( o ) A model for the cell cycle arrest-JNK amplification loop in Ras V12 / mito −/− senescent cells. ( p , q , r ) Adult eye bearing Ras V12 +Hep CA ( p ), Ras V12 +Hep CA +CycE ( q ) or Ras V12 +Hep CA +Catalase ( r ) clones is shown. Scale bars, 50 μm. See Supplementary Table 1 for genotypes. Full size image p53 mediates cell cycle arrest-JNK-dependent SASP Finally, we sought to identify the molecular link between Ras V12 / mito −/− and cell cycle arrest. It has been shown in mouse fibroblasts that the tumour-suppressor gene p53 is required for inducing cell cycle arrest in cells undergoing Ras-induced cellular senescence [42] , [43] , [44] . In addition, it has been shown in Drosophila imaginal disc that p53 and JNK form a positive feedback loop that amplifies their activity/expression [45] . Interestingly, we found that Ras V12 / mito −/− clones strongly upregulate a p53 target gene reaper ( rpr ; Fig. 5a,d ), whereas Ras activation alone or mitochondrial dysfunction alone causes only a moderate or no induction of rpr expression, respectively ( Fig. 5b,c ). Furthermore, Ras V12 / mito −/− clones upregulated p53 expression level ( Fig. 5e,h ), whereas Ras V12 alone or mitochondrial mutation alone caused only a slight upregulation or no upregulation of p53 expression level, respectively ( Fig. 5f,g ). These results indicate that Ras activation and mitochondrial dysfunction cooperate to upregulate p53 activity and raise the possibility that cell cycle arrest in Ras V12 / mito −/− cells is mediated by p53, as previously shown in CoVa −/− clones (cells mutant for mitochondrial respiratory complex IV) [46] . Indeed, removal of p53 in Ras V12 / mito −/− clones significantly suppressed JNK activation (visualized by the mmp1-lacZ reporter [47] ; Fig. 5l , compare with Fig. 5k ) as well as non-autonomous overgrowth ( Fig. 5j , quantified in Supplementary Fig. 5h ). In contrast, removal of p53 did not suppress oxidative stress in Ras V12 / mito −/− clones ( Fig. 5n , compare with Fig. 5m ). In addition, blocking oxidative stress did not suppress upregulation of p53 in Ras V12 / mito −/− clones ( Fig. 5i ), placing p53 in parallel to oxidative stress. These data suggest that elevated p53 activity in Ras V12 / mito −/− cells triggers cell cycle arrest-mediated amplification of JNK signalling, which cooperates with Ras signalling to induce SASP. To test this possibility, we induced clones of cells overexpressing both p53 and Ras V12 in the eye disc and found that these clones indeed induce non-autonomous overgrowth ( Fig. 5o ). Furthermore, the non-autonomous overgrowth caused by Ras V12 +p53 clones was significantly suppressed by JNK inhibition ( Fig. 5p , quantified in Supplementary Fig. 5i ), antioxidant GPx-1 expression ( Fig. 5q , quantified in Supplementary Fig. 5j ), CycE overexpression ( Fig. 5r , quantified in Supplementary Fig. 5k ) and Upd downregulation ( Fig. 5s , quantified in Supplementary Fig. 5l ), suggesting that the overgrowth phenotype was due to SASP. We further confirmed this by immunostaining analyses, which showed that Ras V12 +p53 clones upregulated JNK activity as well as upd expression ( Supplementary Fig. 5a,c,d,f ), whereas clones overexpressing p53 alone caused neither JNK/ upd upregulation ( Supplementary Fig. 5b,e ) nor non-autonomous overgrowth ( Supplementary Fig. 5g ). Altogether, our data indicate that cells with Ras activation and mitochondrial dysfunction lead to production of ROS, downregulation of CycE activity and activation of p53, all of which cooperate together to trigger cell cycle arrest-mediated amplification of JNK signalling and subsequent SASP induction ( Fig. 6 ). 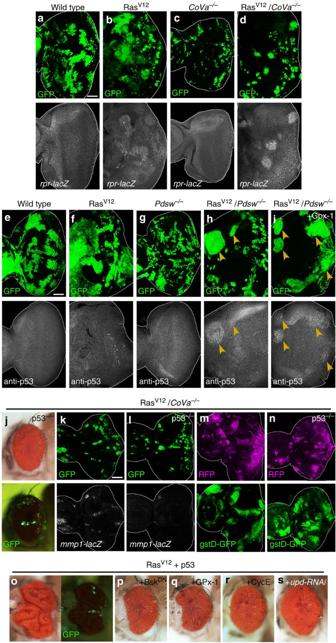Figure 5: p53 mediates cell cycle arrest-JNK-dependent SASP. (a–d) Green fluorescent protein (GFP)-labelled wild-type (a), RasV12(b),CoVa−/−(c) or RasV12/CoVa−/−(d) clones were induced inrpr-lacZeye–antennal disc and stained with anti-β-gal. (e–i) Eye-antennal disc bearing GFP-labelled wild-type (e), RasV12(f),Pdsw−/−(g), RasV12/Pdsw−/−(h) or RasV12/Pdsw−/−+GPx-1 (i) clones was stained with anti-p53 antibody. Arrowheads indicate representative clones upregulating p53. (j) Adult eye bearing GFP-labelled RasV12/CoVa−/−,dmp53−/−clones. (k,l) GFP-labelled RasV12/CoVa−/−(k) or RasV12/CoVa−/−,dmp53−/−(l) clones were induced inmmp1-lacZeye-antennal disc and stained with anti-β-gal. (m,n) RFP-labelled RasV12/CoVa−/−(m) or RasV12/CoVa−/−,dmp53−/−(n) clones were induced ingstD-GFPeye-antennal disc. (o–s) Adult eye bearing RasV12+p53 (o), RasV12+dmp53+BskDN(p), RasV12+dmp53+GPx-1 (q), RasV12+dmp53+CycE (r) or RasV12+dmp53+upd-RNAi(s) clones is shown. Scale bars, 50 μm. SeeSupplementary Table 1for genotypes. Figure 5: p53 mediates cell cycle arrest-JNK-dependent SASP. ( a – d ) Green fluorescent protein (GFP)-labelled wild-type ( a ), Ras V12 ( b ), CoVa −/− ( c ) or Ras V12 / CoVa −/− ( d ) clones were induced in rpr-lacZ eye–antennal disc and stained with anti-β-gal. ( e – i ) Eye-antennal disc bearing GFP-labelled wild-type ( e ), Ras V12 ( f ), Pdsw −/− ( g ), Ras V12 / Pdsw −/− ( h ) or Ras V12 / Pdsw −/− +GPx-1 ( i ) clones was stained with anti-p53 antibody. Arrowheads indicate representative clones upregulating p53. ( j ) Adult eye bearing GFP-labelled Ras V12 / CoVa −/− , dmp53 −/− clones. ( k , l ) GFP-labelled Ras V12 / CoVa −/− ( k ) or Ras V12 / CoVa −/− , dmp53 −/− ( l ) clones were induced in mmp1-lacZ eye-antennal disc and stained with anti-β-gal. ( m , n ) RFP-labelled Ras V12 / CoVa −/− ( m ) or Ras V12 / CoVa −/− , dmp53 −/− ( n ) clones were induced in gstD-GFP eye-antennal disc. ( o – s ) Adult eye bearing Ras V12 +p53 ( o ), Ras V12 +dmp53+Bsk DN ( p ), Ras V12 +dmp53+GPx-1 ( q ), Ras V12 +dmp53+CycE ( r ) or Ras V12 +dmp53+ upd-RNAi ( s ) clones is shown. Scale bars, 50 μm. See Supplementary Table 1 for genotypes. 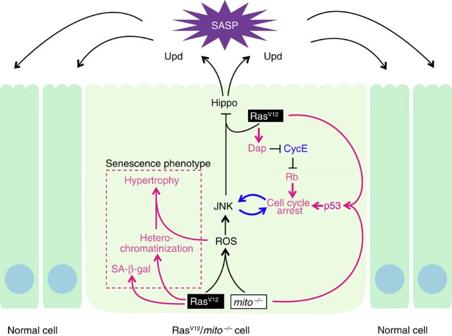Figure 6: A model for the genetic pathway to SASP by Ras activation and mitochondrial dysfunction. Simultaneous Ras activation and mitochondrial dysfunction lead to production of ROS, downregulation of CycE activity and activation of p53, which form the cell cycle arrest-JNK amplification loop. Activated JNK further cooperates with Ras signalling to inactivate the Hippo pathway, leading to upregulation of an inflammatory cytokine Upd. Our data show that mitochondrial defect promotes Ras-induced cellular senescence and thereby contributes to tumour progression of neighbouring tissue through SASP. Full size image Figure 6: A model for the genetic pathway to SASP by Ras activation and mitochondrial dysfunction. Simultaneous Ras activation and mitochondrial dysfunction lead to production of ROS, downregulation of CycE activity and activation of p53, which form the cell cycle arrest-JNK amplification loop. Activated JNK further cooperates with Ras signalling to inactivate the Hippo pathway, leading to upregulation of an inflammatory cytokine Upd. Our data show that mitochondrial defect promotes Ras-induced cellular senescence and thereby contributes to tumour progression of neighbouring tissue through SASP. Full size image Although accumulating evidence has suggested that cell–cell interactions between premalignant cells and senescent cells within tumour microenvironment play important roles in cancer development, the mechanisms underlying such tumour progression have been elusive. In this study, we found in Drosophila imaginal epithelium that Ras activation and mitochondrial dysfunction cooperate to induce cellular senescence, which induces oncogenic SASP through the cell cycle arrest-JNK amplification loop. Our data unveil the genetic pathway of cellular senescence phenotypes such as heterochromatinization, cellular hypertrophy, cell cycle arrest and SASP ( Fig. 6 ). Given that Ras V12 / mito −/− cells are resistant to apoptosis [24] , such senescent cells could exist in tumour tissue for a long period and contribute to tumour progression through chronic ‘oncogenic inflammation’ by SASP factors. In mammalian systems, cellular senescence is caused through p53-mediated cell cycle arrest, which is induced by activation of oncogenes or other cellular stresses such as oxidative stress. Interestingly, we found in Drosophila epithelium that mitochondrial defects in Ras-activated cells trigger ROS production and p53 activation, both of which cooperate to trigger cell cycle arrest-mediated amplification of JNK signalling, a key regulator for SASP induction. Although our data show that p53 is required for the onset of SASP, it has been reported in mammalian systems that p53 is dispensable for SASP or senescence-associated inflammatory response induction [17] , [48] . This discrepancy could be due to the differences in the triggers of cellular senescence (mitochondrial dysfunction, X-irradiation/replicative exhaustion or loss of casein kinase 1 α1) and/or cellular contexts ( in vivo epithelium, cell cultures or organoid cultures) examined in the studies. Our data suggest that in in vivo situations cellular senescence and SASP are triggered or enhanced by additional cellular stresses such as mitochondrial dysfunction in conjunction with Ras activation. Given that mitochondrial respiratory function is frequently downregulated in many types of cancers [49] , similar mechanism of SASP induction could be involved in the progression of Ras-activated human cancers. Studies in mammalian systems have shown that cells undergoing cellular senescence produce SASP factors through nuclear factor-κB signalling or epigenetic control of SASP genes [36] , [50] , [51] . Intriguingly, our genetic study in Drosophila revealed that SASP factors are produced through inactivation of the Hippo pathway, a signalling often deregulated in human cancers [52] . A similar mechanism of SASP induction via the Hippo pathway may also be involved in mammalian tumour tissues with senescent cells. Indeed, a study in mice has shown that the SASP factor IL-6 is significantly upregulated in the liver doubly mutant for mst1 / mst2 (ref. 53 , mammalian orthologues of the hippo gene. Our finding that the cellular senescence machinery also exits in invertebrates suggests that cellular senescence plays a role not only in tumour regulation but also in some evolutionarily conserved physiological contexts such as normal development. Interestingly, it has recently been reported that cellular senescence is required for tissue remodelling during mouse development [54] . Given that Ras signalling, a major trigger for cellular senescence, plays crucial roles in cell proliferation, cell survival, cell differentiation and tissue morphogenesis in both vertebrates and invertebrates, further genetic studies using the Drosophila model may unveil the physiological roles of cellular senescence during normal development and homeostasis. Fly strains and generation of clones Fluorescently labelled mitotic clones [23] were produced in larval imaginal discs using the following strains: y, w, eyFLP1; Act>y + >Gal4, UAS-GFP; FRT82B, Tub-Gal80 (82B tester-1), eyFLP5, Act>y + >Gal4, UAS-GFP; FRT82B, Tub-Gal80 (82B tester-2), y, w, eyFLP1; Act>y + >Gal4, UAS-mmRFP; FRT82B, Tub-Gal80 (82B RFP-tester) , Tub-Gal80, FRT40A, UAS-Ras V12 ; eyFLP6, Act>y + >Gal4, UAS-GFP (40A Ras tester), Tub-Gal80, FRT40A; eyFLP6, Act>y + >Gal4, UAS-GFP (40A tester). Additional strains used were as follows: UAS-Bsk DN (a gift from T. Adachi-Yamada), UAS-Hep, UAS-Hep CA (a gift from T. Adachi-Yamada), UAS-Eiger , CoVa tend , dmp53 [11-1B-1] (a gift from U. Banerjee), mmp1-lacZ (a gift from M. Uhlirova) , rpr-11-lacZ (a gift from J. Abrams), upd-lacZ (a gift from H. Sun), UAS-S/G2/M-Green fucci [26] , UAS-GPx-1 (a gift from F. Missirlis), UAS-CycE, UAS-p35, UAS-dmp53, gstD-GFP (a gift from D. Bormann), Pdsw k10101 , puc E69 , dap k07309 , UAS-Ras V12 , RFP-HP1, UAS- HP1-RNAi , UAS-upd1-RNAi , and UAS- cyclinE-RNAi . Histology Larval tissues were stained with standard immunohistochemical procedures using rabbit anti-Upd polyclonal antibody (1:500; a gift from D. Harrison), rabbit anti-β-galactosidase polyclonal antibody (Sigma, 1:500), mouse anti-phospho-JNK monoclonal antibody G9 (Cell Signaling, 1:100), mouse anti-Dacapo monoclonal antibody NP1 (Developmental Studies Hybridoma Bank, 1:6 for 7 days), mouse anti-BrdU monoclonal antibody BMG 6H8 (Roche, 1:100), rabbit anti-Histone H3 (tri methyl K9) polyclonal antibody (Abcam, 1:50), rabbit anti-RFP antibody (1:500), mouse anti-dmp53 monoclonal antibody p53 7A4 (Developmental Studies Hybridoma Bank, 1:500 for 4 days), mouse anti-γ-H2Av monoclonal antibody UNC93-5.2.1 (ref. 56 ); Developmental Studies Hybridoma Bank, 1:200–400) or Alexa546-conjugated phalloidin (Molecular Probes, 1:50) and were mounted with DAPI-containing SlowFade Gold Antifade Reagent (Molecular Probes). For BrdU labelling, larvae were dissected in Schneider’s medium and incubated in the same media with 10 mM BrdU for 5 min. After incubation with supplied buffer (Roche, 5-Bromo-2′-deoxyuridine labeling and detection kit I) containing 50 U ml −1 DNase I, imaginal discs were stained with anti-BrdU monoclonal antibody BMG 6H8 (Roche, 1:100) and were mounted as descried above. Images were taken with a Zeiss LSM510, Zeiss LSM700 META (Zeiss) or Leica SP5 confocal microscope (Leica). SA-β-gal staining The SA-β-gal activity was visualized using the Senescent Cells Histochemical Staining Kit (CS0030, Sigma-Aldrich). Larvae were dissected in PBS and incubated in the 0.6xStaining Mixture for 90 h at 37 °C. Images were taken with a stereomicroscope. How to cite this article: Nakamura, M. et al. Mitochondrial defects trigger proliferation of neighbouring cells via a senescence-associated secretory phenotype in Drosophila . Nat. Commun. 5:5264 doi: 10.1038/ncomms6264 (2014).